A two-faced selectivity solution to target SMARCA2 for cancer therapy 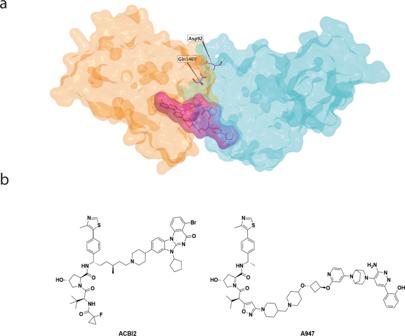Fig. 1: PROTAC-mediated ternary complex formation between SMARCA2 and the E3 ligase, VHL. aA representation of a SMARCA2-PROTAC-VHL ternary complex indicating SMARCA2-exclusive PROTAC-induced interactions (based on PDB: 7Z76, SMARCA2, =orange; PROTAC = purple; VHL = blue).bChemical structures of SMARCA2-selective VHL PROTACs ACBI2 (left) and A947 (right). Now, two recent papers from Kofink et al. and Cantley et al. have prospectively targeted the PROTAC-mediated ternary complex to solve the apparently intractable SMARCA2/4 selectivity problem [12] , [13] . It has been reported previously by Farnaby et al. that potent dual SMARCA2/4 degradation can be achieved using PROTACs derived from ligands targeting the druggable SMARCA2/4 bromodomains rather than the less tractable ATPase domains [14] . While inhibition of the bromodomains fails deliver antiproliferative effects, this is not an issue for a PROTAC where the entire protein is degraded. This ternary complex driven optimisation led to dual PROTAC ACBI1, which replicates the SMARCA2 RNAi phenotype in SMARCA4 deficient cell lines, but does not achieve degradation selectivity for SMARCA2. Kofink et al. build on the identification of ACBI1, with the challenging task of achieving both selective SMARCA2 degradation and oral bioavailability [12] . This started with careful selection of the SMARCA2/4 bromodomain binder to minimise hydrogen bond donors and increase rigidity, which has been shown to improve likelihood of increased oral bioavailability for compounds beyond the rule-of-five [15] . A key aspect of this work was the availability of ternary complex crystal structures which highlighted the proximity of the SMARCA2 bromodomain and VHL binding sites in the complex, indicating that only short linkers would be necessary. This linker exploration identified extraordinarily selective SMARCA2 degraders with the most selective exhibiting >1000-fold degradation selectivity over SMARCA4. This could be rationalised by a ternary crystal structure of a close analogue, indicating a PROTAC-induced protein-protein interaction with SMARCA2 residue Gln1469 which is not conserved in SMARCA4 (Fig. 1a ). Unfortunately, the properties of the highly SMARCA2-selective compounds did not have appropriate physicochemical properties to achieve oral exposure. This emphasises the compromises that must be made in the multi-parameter optimisation of therapeutic PROTACs, as the precise molecular conformation required to achieve ternary complex selectivity may not overlap with the restricted conformations required to achieve oral bioavailability. Fig. 1: PROTAC-mediated ternary complex formation between SMARCA2 and the E3 ligase, VHL. a A representation of a SMARCA2-PROTAC-VHL ternary complex indicating SMARCA2-exclusive PROTAC-induced interactions (based on PDB: 7Z76, SMARCA2, =orange; PROTAC = purple; VHL = blue). b Chemical structures of SMARCA2-selective VHL PROTACs ACBI2 (left) and A947 (right). Full size image Further work exploring extension of the linker between the SMARCA2/4 and VHL binders began to introduce the desired oral bioavailability into the PROTACs, at the expense of some SMARCA2 selectivity. Ultimately this led to the discovery of PROTAC ACBI2 which possess nanomolar degradation potency for SMARCA2, ~30-fold degradation selectivity over SMARCA4 and oral bioavailability of 22% in mouse (Fig. 1b ). When ACBI2 was dosed orally in a SMARCA2-sensitive mouse xenograft model, almost complete degradation of SMARCA2 was achieved although this was associated with tumour stasis rather than the hoped-for regression. The second paper from Cantley et al. describes a structurally distinct and highly potent SMARCA2-selective PROTAC A947 (Fig. 1b ) [13] . In this case, an alternative exit vector from the VHL E3 ligase binder was used, connected to a more advanced SMARCA2/4 ligand, similar to that used previously in ACBI1 [14] . This resulted in extremely potent, sub-nanomolar degradation of SMARCA2 with ~30x selectivity over SMARCA4. In this case, the physicochemical properties of the SMARCA2/4 ligand used in A947 proved to be restrictive to IV dosing. When A947 was administered in SMARCA4-mutant xenograft studies, tumour stasis was again observed despite >95% reduction of SMARCA2 levels in the tumours. Interestingly, it was found that selective degradation of SMARCA2 could be achieved with partial sparing of SMARCA4, consistent with the selectivity profile observed in vitro, indicating the potential for SMARCA2 degradation selectivity by appropriate dose selection. Given SMARCA2 degradation failed to meet expectations for tumour efficacy, combinations were explored, which led to identification of in vitro sensitisation to apoptosis through combination with MCL1 inhibitors. Both papers demonstrate the unique benefit of PROTACs both in the utilisation of non-functionally relevant binding sites and critically for achieving selectivity through complementary ternary complex formation, delivering selective pharmacological SMARCA2 degradation. In both cases, the SMARCA2-SMARCA4 synthetic lethal relationship was validated in vivo and built on the existing in vitro evidence. Others looking to solve intractable selectivity challenges will no doubt be inspired by these results, and we can expect to see further examples of this strategy appearing in the literature in the future.